The biology and chemistry of high-valent iron–oxo and iron–nitrido complexes High-valent oxoiron(IV) and formally oxoiron(V) species have been spectroscopically identified as active intermediates in the catalytic cycles of a number of enzymatic systems [1] , [2] , [3] , [4] , [5] , [6] , [7] , [8] , [9] , [10] . Haem and non-haem proteins use these reactive intermediates to couple the activation of dioxygen to the oxidation of their substrates. In most cases, an oxygen atom is inserted into an unactivated C–H bond of the substrate; for example, in hydroxylation reactions [1] , [2] , [3] , [4] , [5] , [6] , [7] , [8] , [9] , [10] . However, many other reactions, including halogenation, desaturation, cyclization, epoxidation and decarboxylation, are also known to involve oxoiron species [1] , [3] . Superoxidized iron complexes with (valence) isoelectronic imido and nitrido ligands, as well as 'surface nitrides', have also been implicated as key intermediates in the nitrogen atom transfer reactions [11] , the biological synthesis of ammonia by the nitrogenase enzyme [12] , [13] , [14] , [15] , [16] and the industrial Haber-Bosch process [17] . The generation of well-described model compounds can provide vital insights into the mechanism of such enzymatic reactions. Consequently, considerable effort has been made by synthetic chemists to prepare viable models for the putative reaction intermediates in the catalytic cycles of O 2 and N 2 activating enzymes. In this review, we provide an overview of all high-valent oxoiron and nitridoiron species that have been either identified or proposed as reactive intermediates in biology. Subsequently, we summarize some of the recent advances in bioinorganic chemistry that have led to the identification and isolation of iron complexes in unusually high formal oxidation states, containing iron–oxygen or iron–nitrogen multiple bonds. The spectroscopic characterization and the reactivity studies of these model complexes provide vital insights into the mechanism that nature uses to induce the reductive cleavage of dioxygen or dinitrogen in carrying out a number of important biochemical oxidative transformations. Moreover, the comparative review of the electronic structures of the isoelectronic oxoiron and nitridoiron functionalities reveals that the Fe–N bonds are intrinsically more covalent than the Fe–O bonds. Iron–oxo intermediates in biology Heme and non-heme proteins activate dioxygen or hydrogen peroxide to generate high-valent oxoiron reactive intermediates, which are used to carry out a diverse set of biological tasks [1] , [2] , [3] , [4] , [5] , [6] , [7] , [8] , [9] , [10] . Important processes such as catabolism, angiogenesis, respiration, and apoptosis rely on oxidation reactions driven by these reactive intermediates [1] , [2] , [3] . The coordination environment of the oxoiron unit is, however, found to be different in different enzymes. Three types of high-valent iron–oxo active sites have been identified in haem and non-haem enzymes ( Fig. 1 ). The haem-containing peroxidases, oxygenases and catalases comprise mononuclear iron-protophyrin IX active sites coordinated to either a cysteine, histidine or tyrosine residue [3] , [18] . The second type involves mononuclear iron centres that are coordinated to two histidines and a carboxylate group, thereby forming a characteristic 2-His-1-carboxylate facial triad, which has been recognized as a common structural motif for many mononuclear non-haem iron enzymes [1] , [2] , [3] . The third type of active sites is characterized by diiron centres with two histidines and four carboxylates and are associated with methane and toluene monooxygenases, fatty acid desaturases and ribonucleotidereductase [5] , [10] . Most of these enzymes activate dioxygen in the iron(II) state and carry out a variety of two-electron oxidation processes ( Fig. 2 ); the remaining two reducing equivalents required for the four-electron reduction of dioxygen are often provided by a cosubstrate ( Fig. 1 ). One specific group of non-haem enzymes utilizes 2-oxoacids or tetrahydrobiopterin as the cosubstrate, delivering two electrons simultaneously to the active site to afford peroxoiron(II) and oxoiron(IV) species in the proposed reaction mechanism [1] . Enzymes, such as cytochrome-P450 (P450), soluble methane monooxygenase (sMMO) or Rieske dioxygenases, on the other hand, use NADH as the electron donor to form peroxoiron(III) and formally oxoiron(V) species ( Fig. 1 ); all the redox equivalents of the formal oxoiron(V) species are stored either at the metal centre(s) in non-haem enzymes (for example, Fe 2 IV (μ-O) 2 intermediate Q in sMMO [5] , [10] and (OH)Fe V =O intermediate [4] in Rieske dioxygenase) or distributed over the ligand in haem enzymes (for example, Compound-I (Cpd-I), which is an oxoiron(IV) porphyrin π-cation radical species) [3] , [6] , [7] , [9] . In addition to dioxygen, hydrogen peroxide can also act as an oxygen-atom source by reacting directly with the iron(III) state of the enzyme [3] , [6] , [9] , to generate the active oxidant (no reductase components are required in this case). 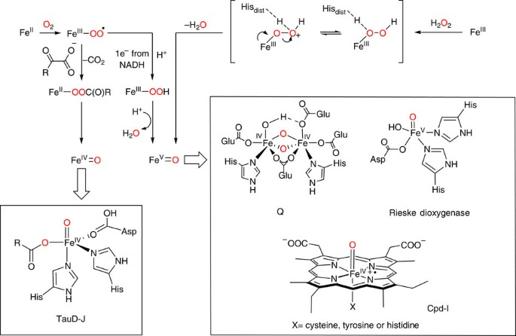Figure 1: Mechanisms of dioxygen and hydrogen peroxide activation by iron containing haem and non-haem oxygenases. The structures in the boxes depict high-valent intermediates of the enzymatic reactions; TauD-J: intermediate J of taurine dioxygenase, Q: intermediate Q of soluble methane monooxygenase, Cpd-I: Compound-I intermediates of iron containing haem enzymes, like catalase, peroxidase or cytochrome-P450; His: histidine; Hisdist: distal histidine; Asp: asparagine; Glu: glutamic acid. Figure 1: Mechanisms of dioxygen and hydrogen peroxide activation by iron containing haem and non-haem oxygenases. The structures in the boxes depict high-valent intermediates of the enzymatic reactions; TauD-J: intermediate J of taurine dioxygenase, Q: intermediate Q of soluble methane monooxygenase, Cpd-I: Compound-I intermediates of iron containing haem enzymes, like catalase, peroxidase or cytochrome-P450; His: histidine; His dist : distal histidine; Asp: asparagine; Glu: glutamic acid. 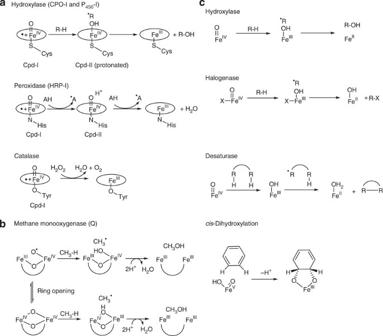Figure 2: Reactions catalysed by high-valent oxo intermediates of iron-containing enzymes. Enzyme reactions: (a) haem enzymes, (b) a non-haem diiron enzyme and (c) non-haem monoiron enzymes. Cpd-I, compound-I of iron containing haem enzymes; Cpd-II, compound-II of iron containing haem enzymes; CPO-I, compound-I of chloroperoxidase; P450-I, compound-I of cytochrome-P450; HRP-I, compound-I of horse-radish peroxidase; AH, reducing substrate for peroxidase (in case of glutathione peroxidase AH is monomeric glutathione); Cys, cysteine; Tyr, tyrosine. Full size image Figure 2: Reactions catalysed by high-valent oxo intermediates of iron-containing enzymes. Enzyme reactions: ( a ) haem enzymes, ( b ) a non-haem diiron enzyme and ( c ) non-haem monoiron enzymes. Cpd-I, compound-I of iron containing haem enzymes; Cpd-II, compound-II of iron containing haem enzymes; CPO-I, compound-I of chloroperoxidase; P450-I, compound-I of cytochrome-P450; HRP-I, compound-I of horse-radish peroxidase; AH, reducing substrate for peroxidase (in case of glutathione peroxidase AH is monomeric glutathione); Cys, cysteine; Tyr, tyrosine. Full size image These high-valent iron–oxo intermediates in biology have been primarily characterized by 57 Fe Mössbauer spectroscopy [19] , as it serves as a local probe of the iron centre. Mössbauer isomer shifts ( δ ) are directly related to the electron density at the iron nucleus and, therefore, are often used as a probe of the 'oxidation state' of the metal. The quadrupole splitting (Δ E Q ) values, on the other hand, are a measure of the electric field gradient at the iron nucleus and can be strongly correlated to electronic spin ground state and molecular geometry. Nuclear hyperfine tensors (A) depend strongly on the nature of the orbitals in which unpaired electrons reside and may be used as a tool to understand the electronic structure of paramagnetic species. Whereas δ and Δ E Q values ( Table 1 ) obtained from zero-field Mössbauer studies of the active oxidants in both haem and non-haem oxygenases are consistent with an iron(IV) oxidation state, the analysis of the Mössbauer spectra in an applied magnetic field reveals different spin states in the two cases. For haem enzymes the A tensor shows a qualitative trend of 'two large negative values, one small negative value' [20] , [21] , thereby reflecting an intermediate spin, S =1 spin state for the iron(IV) centre. In CPd-I intermediates, this S =1 spin state is coupled ferromagnetically or antiferromagnetically to the porphyrin radical cation, giving an overall quartet or doublet state, respectively [3] , [6] , [7] , [9] . In contrast, for the non-haem case, a high-spin S =2 state is demonstrated by 'three large negative' A tensors [1] , [19] . The high-spin configuration is possibly due to the weak ligand field exerted by the combination of histidine and carboxylate ligands or the proposed pseudo-trigonal symmetry [22] , which renders the d ( x 2 − y 2 ) and d ( xy ) orbitals nearly degenerate in energy ( Fig. 3 (refs 23 and 24 )). Table 1 Structural and spectroscopic properties of high-valent iron–oxo and –nitrido units in chemistry and biology. 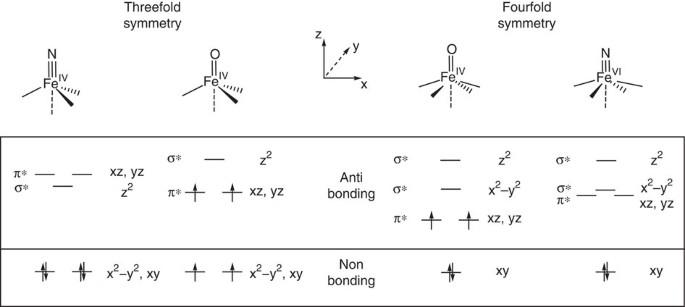Figure 3: Tetragonal and trigonal ligand fields of high-valent transition metal complexes with strong σ-donor oxo and nitrido ligands23,24. In threefold symmetry, a non-bonding, doubly degenerate set of (x2–y2,xy) orbitals allows for the stabilization and isolation of nitridoiron(IV) and (V) complexes and enables the spin stateS=2 for oxoiron(IV) species. In tetragonal ligand fields, oxo complexes exhibit the classical 1+2+1+1d-orbital energy scheme (ref.49). According to Bendixet al. (ref.23), complexes with the more covalent nitrido and weak equatorial ligands deviate from this and approach a 1+3+1 splitting diagram, in which thex2−y2orbital can even be lower in energy than the (xz,yz) set. Full size table Figure 3: Tetragonal and trigonal ligand fields of high-valent transition metal complexes with strong σ-donor oxo and nitrido ligands [23] , [24] . In threefold symmetry, a non-bonding, doubly degenerate set of ( x 2 – y 2 , xy ) orbitals allows for the stabilization and isolation of nitridoiron(IV) and (V) complexes and enables the spin state S =2 for oxoiron(IV) species. In tetragonal ligand fields, oxo complexes exhibit the classical 1+2+1+1 d -orbital energy scheme (ref. 49 ). According to Bendix et al . (ref. 23 ), complexes with the more covalent nitrido and weak equatorial ligands deviate from this and approach a 1+3+1 splitting diagram, in which the x 2 − y 2 orbital can even be lower in energy than the ( xz , yz ) set. Full size image In spite of the spin state difference in the mononuclear high-valent oxoiron(IV) intermediates of the haem and non-haem enzymes, the Fe–O bond strengths for the S =1 and S =2 states are comparable. The Fe=O bond distances (1.64–1.68 Å), obtained from extended X-ray absorption fine structure (EXAFS) or X-ray diffraction studies, and the Fe–O stretching frequencies (776–843 cm −1 ), obtained from resonance Raman studies, are found to be similar in both cases [1] , [2] , [3] , [5] , [6] , [7] , [9] , [10] , [18] . This similarity is expected based on the molecular orbital diagram shown in Fig. 3 . For both the S =1 and S =2 configurations the Fe–O antibonding π*{( d ( xz ), d ( yz )} levels contain two electrons. A significantly larger Fe–O distance (1.81 Å) and lower Fe–O stretching frequency (565 cm −1 ), however, are observed for the one-electron reduced form of Cpd-I of the thiolate-ligated haem enzymes, where the oxoiron(IV) unit is protonated ( Fig. 2 ) [25] , [26] , [27] , [28] . A protonated oxoiron(IV) centre is also reflected in the Mössbauer data as the variation of the Fe d ( xz )/ d ( yz ) spin populations, owing to the protonation of the oxoiron(IV) unit, provides unique Δ E Q values significantly larger (>2 mm s −1 ) than those in the deprotonated form (<1.6 mm s −1 ) [25] , [26] , [27] , [28] . Iron–oxo model complexes The first high-valent oxoiron complex was synthesized in 1981 by Groves et al . [7] , [8] via oxidation of [(TMP)Fe III (Cl)] (TMP=meso-tetramesityl porphinate anion) with meta-chloroperbenzoic acid in a dichloromethane-methanol mixture at −78 °C. On the basis of its absorption spectra, the electronic structure of the resultant green compound was best described as an oxoiron(IV) porphyrin π-radical cation (d 4 ) species [(TMP +• )Fe IV (O)(CH 3 OH)] + , which showed the characteristic features of Cpd-I intermediates; namely, a weak and broad Soret band at 405 nm and a Q-band at 605 nm [6] , [9] . On the basis of electron paramagnetic resonance (EPR) and applied-field Mössbauer spectroscopy ( Table 1 ), an overall quartet ( S t =3/2) ground state was deduced, arising from a ferromagnetic coupling of the S =1 iron(IV) centre with a porphyrin π-cation radical ( S =1/2). The structural analysis of the intermediate by EXAFS revealed a short Fe–O bond distance of 1.60 Å, indicating that Fe=O possesses double-bond character. The oxoiron(IV) double-bond character is further supported by a resonance Raman vibrational band centred at ν =828 cm −1 in dichloromethane methanol, which was assigned to the ν (Fe–O) stretching vibration based on its shift to 792 cm −1 on 18 O labelling. In the absence of methanol, the ν (Fe–O) stretching vibration was observed at 801 cm −1 due to the binding of the chloride anion as an axial ligand trans to the oxo unit. Thus, as also suggested from theoretical studies [29] , the axial ligand competes with the oxo-group in binding to the iron-centre, therefore decreasing the strength of the Fe–O bond. The [(TMP +• )Fe IV (O)(CH 3 OH)] + complex was found to be a competent oxidant in olefin epoxidation and alkane hydroxylations [6] , [7] . Since then, a number of oxoiron(IV) porphyrin π-radicals bearing electron-rich and -deficient porphyrins ( Fig. 4 ) have been prepared in an effort to understand the electronic effects of the porphyrins on the chemical properties of the oxoiron(IV) intermediates [3] . The results of these studies, which are summarized in some recent review articles [3] , [6] , [7] , indicate that the electronic nature of porphyrin ligands controls the oxidizing power of oxoiron porphyrins, and that oxoiron species with electron-deficient porphyrins are more powerful oxidants in the oxygenation of organic substrates. The axial ligands bound trans to the iron–oxo moiety also markedly influence the reactivities of oxoiron(IV) porphyrin π-cation radicals. For example, a recent study by Kang et al . [30] , which investigated a series of complexes [(TMP +• )Fe IV (O)( p -Y-pyO)] + (Y=OCH 3 , CH 3 , H, Cl) and [(TMP +• )Fe IV (O)(X)] (X=CF 3 SO 3 − , Cl − , AcO − , OH − ) in H-atom abstraction and O-transfer reactions by experimental ( Fig. 5a ) and theoretical methods, showed that rates of both the O-transfer and H-atom abstraction reactions of the porphyrin complexes increase with increasing electron donation from the axial ligand. Their results have been extended to correlate the strong oxidizing power of the thiolate-ligated P450 enzyme to the strong electron donation from the axial thiolate ligand [31] . 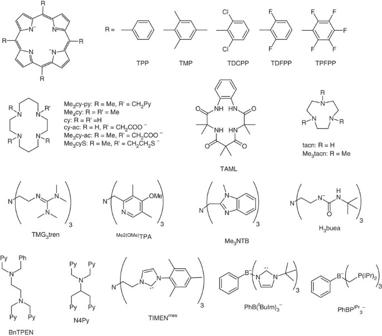Figure 4: Macrocyclic and chelating ligands for the stabilization of high-valent oxo– and nitrido–iron complexes. Structures in the first line depict porphyrin-based ligands; in the second line macrocyclic ligands, involving amine or amide nitrogen donors; in the third and fourth line, nitrogen- and boron-anchored tri- and tetrapodal chelates. Py, 2-pyridyl group; Ph, phenyl group;iPr,iso-propyl group. Figure 4: Macrocyclic and chelating ligands for the stabilization of high-valent oxo– and nitrido–iron complexes. Structures in the first line depict porphyrin-based ligands; in the second line macrocyclic ligands, involving amine or amide nitrogen donors; in the third and fourth line, nitrogen- and boron-anchored tri- and tetrapodal chelates. Py, 2-pyridyl group; Ph, phenyl group; i Pr, iso -propyl group. 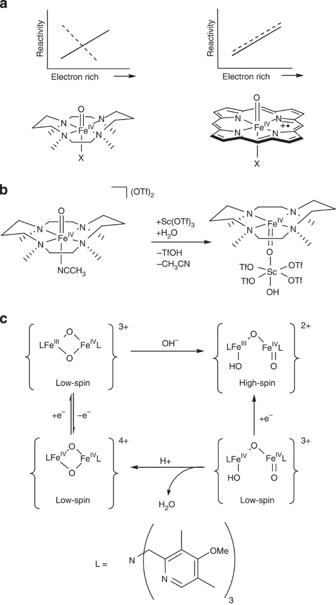Figure 5: Reactivity of high-valent mono- and diiron-oxo model complexes. (a) Axial ligand effects on the oxo-transfer (dotted line) and H-atom abstraction (bold line) reactivity of the complexes [(Me4cy)FeIV(O)X]+(X = NCCH3, −O2CCF3, −N3, or −SR)65and [(TMP)+•FeIV(O)X] (X = CF3SO3−, Cl−, AcO−, OH−)30; (b) Structural changes of the oxoiron(IV) unit of the model complex as a result of binding to a Sc3+ion43; OTf, triflate. (c) Interconversions among high-valent diiron complexes71,73,74. Full size image Figure 5: Reactivity of high-valent mono- and diiron-oxo model complexes. ( a ) Axial ligand effects on the oxo-transfer (dotted line) and H-atom abstraction (bold line) reactivity of the complexes [(Me 4 cy)Fe IV (O)X]+(X = NCCH 3 , −O2CCF 3 , −N 3 , or −SR) [65] and [(TMP) +• Fe IV (O)X] (X = CF 3 SO 3 −, Cl−, AcO−, OH−) [30] ; ( b ) Structural changes of the oxoiron(IV) unit of the model complex as a result of binding to a Sc 3+ ion [43] ; OTf, triflate. ( c ) Interconversions among high-valent diiron complexes [71] , [73] , [74] . Full size image In contrast to the haem-based systems, which mainly stabilize an oxoiron(IV) π-cation radical unit, an iron(V) oxidation state can be stabilized with redox-innocent, non-haem ligand systems. Accordingly, Tiago de Oliveira et al . [32] reported the synthesis of an oxoiron(V) (d 3 ) complex by using their signature tetraamido macrocyclic ligand (TAML). The reaction of [(TAML)Fe III (H 2 O)] − with meta-chloroperbenzoic acid in n -butyronitrile at −60 °C, in presence of small amounts of water, pyridine or benzoic acid, yielded a deep green complex, which has been characterized as [(TAML)Fe V (O)] − , based on a combined Mössbauer, EPR and EXAFS study. The iron(V) oxidation state was confirmed on the basis of its characteristic Mössbauer spectrum with an unusually low, negative isomer shift of −0.42 mm s −1 and large quadrupole splitting of 4.25 mm s −1 at 4.2 K ( Table 1 ). The EPR spectrum revealed an S =1/2 ground state, and EXAFS provided evidence of a short Fe–O distance of 1.58 Å consistent with the [(TAML)Fe V (O)] − assignment for the complex. An Fe V (O)(OH) species has been implicated as the active oxidant responsible for the cis -dihydroxylation of C=C double bonds [2] , [4] , [33] and the oxidation of water [34] in a number of iron-containing non-haem natural and model systems, but with only indirect proof of its existence [35] , [36] , [37] . However, the spectroscopically characterized [(TAML)Fe V (O)] − anion, which is the only known isolable oxoiron(V) species in the literature, was found to be a sluggish oxidant [32] ; reacting with the weak C–H bonds of dihydroanthracene only. Moreover, no [(TAML)Fe V (O)] − mediated cis -dihydroxylation reaction have thus far been reported. Additionally, no [(TAML)Fe V (O)] − intermediate could be identified during the [(TAML)Fe III ] − mediated water oxidation reaction [38] . Therefore, the involvement of Fe V (O)(OH) intermediates in oxygenation reactions remained doubtful until very recently [39] . Using variable-temperature mass spectrometry, Prat et al . [39] provided evidence for such a reactive intermediate in a synthetic system. While the first paper on the synthesis and characterization of an oxoiron(IV) porphyrin species appeared in 1981 (ref. 8 ), the original report of a non-haem oxoiron(IV) complex appeared almost two decades later in 2000 (ref. 40 ). The biggest impediment to progress in identifying and trapping a non-haem oxoiron(IV) species was the lack of a convenient spectroscopic signature that would readily signal its presence in a reaction mixture. Although oxoiron(IV) porphyrin complexes had been well characterized for some time, their ultraviolet–visible spectra were dominated by intense porphyrin ligand transitions that obscured weaker bands that may be associated with the Fe IV =O unit. Thus, design of suitable ligand systems to stabilize oxoiron(IV) units in non-haem ligand environment was warranted so as to obtain deeper insights into their electronic structure. Grapperhaus et al . [40] were the first to obtain a major breakthrough in this regard. They generated a terminal non-haem oxoiron(IV) species by the ozonolysis of [(cy-ac)Fe III (CF 3 SO 3 )] + (cy-ac=1,4,8,11-tetraazacyclotetradecane-1-acetate) in a mixture of acetone/water at −80 °C. The fleeting intermediate was characterized to be a low-spin ( S =1) iron(IV) species based on Mössbauer studies ( δ =0.1 mm s −1 and Δ E Q =1.39 mm s −1 ) [40] . The instability of the compound, however, prevented its further spectroscopic characterization. Subsequently, Rohde et al . [41] reported the first X-ray crystal structure of a mononuclear S =1 oxoiron(IV) complex that was generated in the reaction of [(Me 4 cy)Fe II (CH 3 CN)] 2+ (Me 4 cy=1,4,8,11-tetramethylcyclam) and iodosobenzene (PhIO) in CH 3 CN at 25 °C. The molecular structure of the [(Me 4 cy)Fe IV (O)(CH 3 CN)] 2+ complex features a short Fe=O distance of 1.646(3) Å with an acetonitrile ligand bound trans to the oxo group ( Fig. 5b ). The macrocyclic Me 4 cy ligand adopts a trans -I configuration [42] such that all four methyl groups are oriented anti to the oxo atom. A syn orientation of the oxo group has also been recently demonstrated in the crystal structure of the [(Me 4 cy)Fe IV (O)Sc(OSO 2 CF 3 ) 4 OH] complex, formed by the reaction of [(Me 4 cy)Fe IV (O)(CH 3 CN)] 2+ with Sc(CF 3 SO 3 ) 3 [43] . In addition to the oxo-ligand inversion, the strong binding of Sc 3+ to the Fe=O moiety of the [(Me 4 cy)Fe IV (O)(CH 3 CN)] 2+ complex induces a pentacoordinated square-pyramidal coordination at the iron centre and an elongated Fe–O distance of 1.754(3) Å. Since the report of the [(Me 4 cy)Fe IV (O)(CH 3 CN)] 2+ complex in 2003, a handful of non-haem S =1 oxoiron(IV) complexes have been synthesized in the past 8 years, using various tetradentate and pentadentate ligand systems ( Fig. 4 ), containing pyridine and amine nitrogen donors [33] , [44] . The structural analysis of the intermediates by X-ray crystallography for [(Me 4 cy)Fe IV (O)(CH 3 CN)] 2+ , [(Me 3 cy-py)Fe IV (O)] 2+ (Me 3 cy-py=1-(2′-pyridylmethyl)-4,8,11-trimethyl-1,4,8,11-tetraazacyclotetradecane) [45] and [(N4Py)Fe IV (O)] 2+ (N4Py= N,N -bis(2-pyridylmethyl)-bis(2-pyridyl)methylamine), or EXAFS for others, revealed a short Fe–O distance of ∼ 1.64 Å, which is comparable with those of oxoiron(IV) porphyrin intermediates [6] , [7] , [9] , [18] and significantly different from the 1.81 Å distance of Borovik's oxoiron(III) [46] , 1.75 Å of Nam's [43] [(Me 4 cy)Fe IV (O)Sc(OSO 2 CF 3 ) 4 OH] and the 1.58 Å distance of Collins' oxoiron(V) complexes [32] . Another relatively long Fe–O distance of 1.70 Å has been obtained for the thiolate-ligated [(Me 4 cyS)Fe IV (O)] + (Me 4 cyS=monoanion of 1-(mercaptoethyl)-4,8,11-trimethyl-1,4,8,11-tetraazacyclotetradecane) complex [47] , which acts as the model complex for the recently characterized [48] thiolate-ligated Cpd-I intermediate in the catalytic cycle of P450. All these compounds feature a near-infrared absorption band of moderate intensity [44] , which, on the basis of magnetic circular dichroism, has been attributed to three of the five ligand-field transitions expected for an S =1 Fe(IV) centre in C 4V symmetry [49] . The general method of synthesizing the non-haem oxoiron(IV) complexes involves the reaction of the iron(II) precursor with an oxygen atom donor, like PhIO or peracids ( Fig. 6 ) [44] . In rare cases, they have been generated electrochemically [50] or photochemically [51] , using water as the oxygen source and also by using hydrogen peroxide in presence of a base [52] . Only recently, dioxygen has been used as an oxidant, which has helped to improve our understanding of the mechanism of dioxygen activation at a mononuclear iron active site [45] , [53] , [54] , [55] . Most of the intermediates shown in Fig. 1 have been independently identified and have established the credibility of the proposed mechanism of dioxygen activation. The formation of the high-valent iron oxidant via a reductive O–O bond cleavage step requires two electrons and protons. Thibon et al . [45] used BPh 4 − (electron donor) and HClO 4 (proton donor) to demonstrate the formation of a high-valent S =1 iron(IV) species in [(Me 3 cy-py)Fe IV (O)] 2+ from [(Me 3 cy-py)Fe II ] 2+ and dioxygen. Lee et al . [55] , on the other hand, were able to generate S =1 [(Me 4 cy)Fe IV (O)(CH 3 CN)] 2+ from [(Me 4 cy)Fe II (CH 3 CN)] 2+ and O 2 , using olefins containing allylic C–H bonds as H-atom (H + + e − ) donors. In both studies, no intermediates could be trapped during oxoiron(IV) formation. Hong et al . [53] also reported the synthesis of the known [(N4Py)Fe III -OOH] 2+ or [(BnTPEN)Fe III -OOH] 2+ (BnTPEN= N -benzyl- N,N',N' -tris(2-pyridylmethyl)-1,2-diaminoethane) complexes in near-quantitative yield, by activating dioxygen in the presence of acid and 1-benzyl-1,4-dihydronicotinamide, an NADH analogue. However, no oxoiron(IV) complex could be identified in these reactions as well. The missing link connecting the mechanistic steps of the above studies was the experimental demonstration of O–O bond cleavage in a hydroperoxoiron(III) complex to yield the corresponding high-valent iron–oxo species. This link has recently been identified independently by the groups of Li et al . [56] and Cho et al ., who generated a high-spin Fe III -OOH complex supported by the Me 4 cy ligand via protonation of the side-on peroxoiron(III) conjugate base [56] , [57] . This hydroperoxo complex was shown to convert quantitatively to the corresponding S =1 oxoiron(IV) complex either through acid-mediated O–O bond heterolysis, followed by the reduction of the transient oxoiron(V) intermediate [56] or directly by O–O bond homolysis [57] . 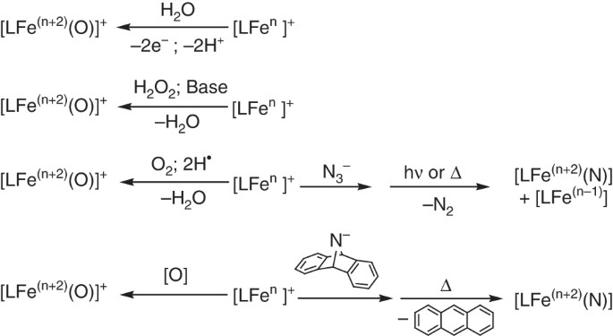Figure 6: Synthetic routes for high-valent oxo– and nitrido–iron complexes. Common synthetic routes for iron–oxo complexes include oxidation of the iron centre with water as an oxygen source50,51or the oxidation of the complex with hydrogen peroxide52,55,56,57, elemental oxygen45,54or other oxygen-atom donors44,47. A number of transition metal nitrido complexes have been synthesized via deoxygenation of NO, reductive decarbonylation of isocyanate,N–Nbond cleavage in N2O reduction, inter-metal N-atom transfer from nitrido complexes, and metathesis of nitrile from metal alkylidyne and a M–M multiple bonded complex. In contrast, fewer synthetic routes are known for iron–nitrido complexes: the photo- and thermolysis of azide precursors80,81, N-atom transfer via strain release by anthracene elimination from 2,3:5,6-dibenzo-7-azabicyclo[2.2.1]hepta-2,5-diene85, and, only recently, with elemental dinitrogen (synthesis not depicted)100. [O] represents oxygen-atom donors, like iodosobenzene or peracids. Figure 6: Synthetic routes for high-valent oxo– and nitrido–iron complexes. Common synthetic routes for iron–oxo complexes include oxidation of the iron centre with water as an oxygen source [50] , [51] or the oxidation of the complex with hydrogen peroxide [52] , [55] , [56] , [57] , elemental oxygen [45] , [54] or other oxygen-atom donors [44] , [47] . A number of transition metal nitrido complexes have been synthesized via deoxygenation of NO, reductive decarbonylation of isocyanate, N – N bond cleavage in N 2 O reduction, inter-metal N-atom transfer from nitrido complexes, and metathesis of nitrile from metal alkylidyne and a M–M multiple bonded complex. In contrast, fewer synthetic routes are known for iron–nitrido complexes: the photo- and thermolysis of azide precursors [80] , [81] , N-atom transfer via strain release by anthracene elimination from 2,3:5,6-dibenzo-7-azabicyclo[2.2.1]hepta-2,5-diene [85] , and, only recently, with elemental dinitrogen (synthesis not depicted) [100] . [O] represents oxygen-atom donors, like iodosobenzene or peracids. Full size image The [(H 3 buea)Fe II ] − complex of the tris(ureaylato) ligand, used by MacBeth et al . [46] , also reacts with O 2 to yield an oxoiron(III) intermediate, which is proposed to derive from the reduction of an initially formed oxoiron(IV) species. Although the oxoiron(IV) species on the way to the generation of the oxoiron(III) complex could not be trapped, it has recently been synthesized by the one-electron oxidation of the preformed [(H 3 buea)Fe III (O)] 2− (ref. 54 ). Interestingly, an S =2 state has been determined for [(H 3 buea)Fe IV (O)] − on the basis of a sharp resonance at g =8.19 in the parallel mode EPR spectra, which is indicative of a transition from the |±2> doublet of an S= 2 spin manifold. Anionic [(H 3 buea)Fe IV (O)] − represents the only example of an S =2 oxoiron(IV) complex generated by O 2 activation. Two examples of synthetic high-spin oxoiron(IV) species have been described before the report of MacBeth et al . (ref. 46 ): one from Pestovsky et al . [58] , using [Fe II (H 2 O) 6 ] 2+ and ozone in water and the other from England et al . [59] , [60] , using [Fe II (TMG 3 tren)(OTf)] + and iodosylbenzene. The S =2 ground state in [(TMG 3 tren)Fe IV (O)] 2+ and [(H 2 O) 5 Fe IV (O)] 2+ has been determined by applied-field Mössbauer studies, which, similar to the oxoiron(IV) intermediates observed in the catalytic cycle of non-haem oxygenases, are characterized by a large and negative hyperfine splitting component in z -direction and by a small and negative quadrupole splitting (Δ E Q ) parameter ( Table 1 ). The molecular structures of [(TMG 3 tren)Fe IV (O)] 2+ and [(H 3 buea)Fe IV (O)] − , as determined by X-ray crystallography, reveal a trigonal bipyramidal geometry at the metal centre, with Fe=O distances of 1.661(2) [60] and 1.680(1) Å [54] , respectively. The S =2 ground state in [(TMG 3 tren)Fe IV (O)] 2+ and [(H 3 buea)Fe IV (O)] − is attributed to their threefold symmetry with degenerate sets of d ( xy ) and d ( x 2 − y 2 ) orbitals ( Fig. 3 ) [23] , [24] . The reactivity of non-haem oxoiron(IV) complexes in C–H hydroxylation and oxo-transfer reactions has been considered in depth by theoretical [61] , [62] , [63] and experimental methods [44] , [64] , [65] . So far, all theoretical studies have led to the common conclusion that the ferryl species are better oxidants on the quintet-state than the corresponding triplet-state. There is a long-term debate, however, on how to rationalize the higher reactivity of the quintate state [66] , [67] , [68] , [69] . Moreover, direct experimental evidence for the higher reactivity of the S =2 state is lacking in the literature. Presumably, because the oxoiron(IV) core is protected by the sterically bulky chelator in the recently reported S =2 [(TMG 3 tren)Fe IV (O)] 2+ complex [59] , [60] , [67] , its reactivity towards C–H bond cleavage is only comparable with triplet ferryl analogues. Indirect evidence of the higher reactivity of the quintate state is, however, provided by Seo et al . [64] in their report of a highly reactive mononuclear oxoiron(IV) complex, [(Me 3 NTB)Fe IV (O)(CH 3 CN)] 2+ (with Me 3 NTB=tris(( N -methyl-benzimidazol-2-yl)methyl)amine), that attacks the strong C–H bonds of cyclohexane at −40 °C. This complex is the most reactive species among oxoiron(IV) complexes reported so far. Although an S =1 ground state has been obtained for the complex from applied-field Mössbauer spectroscopy at 4.2 K, density–functional theory (DFT) calculations explain the unprecedented high reactivity of [(Me 3 NTB)Fe IV (O)(CH 3 CN)] 2+ on the basis of the easily accessible extremely low-lying excited S =2 state that mediates the reactivity. The two-state reactivity, proposed for [(Me 3 NTB)Fe IV (O)(CH 3 CN)] 2+ , has also been used to explain the reactivity pattern of a series of [(Me 4 cy)Fe IV (O)(X)]+ complexes (X=NCCH 3 , − O 2 CCF 3 , − N 3 or − SR) [65] . In this series, the reactivity rates of O-transfer to PPh 3 were found to decrease in the order NCCH 3 > − O 2 CCF 3 > − N 3 > − SR consistent with the decreasing electrophilicity of the Fe=O unit. The rates of H-atom abstraction from dihydroanthracene, however, increased with the introduction of a more electron donating axial ligand ( Fig. 5a ). The latter counter-intuitive trend has been rationalized by the decrease in calculated energy gap between the triplet ground state and the quintet excited state as the axial ligand becomes more electron donating, thereby lowering the activation barrier for H-atom abstraction. This is in contrast to the Cpd-I model compounds (formally oxoiron(V) species), where the determined rates of O-transfer and C–H abstraction reactions increase with increasing donation from the axial ligands ( Fig. 5a ). Dinuclear bis(μ-oxo)diiron(IV) model complexes Intermediate Q is considered as the key oxidizing species in the catalytic cycle of sMMO, performing the chemically exceedingly challenging conversion of methane to methanol. A detailed analysis of EXAFS and Mössbauer spectroscopic data revealed that Q is best described as a strongly exchange-coupled S =2 diiron(IV) species with an Fe–Fe distance of 2.46 Å and pairs of short and long Fe–O bonds of 1.77 and 2.05 Å, respectively, consistent with an Fe 2 IV (μ-O) 2 -diamond core structure [70] . Xue et al . [71] succeeded in preparing the first and only example of a synthetic complex possessing a Fe 2 IV (μ-O) 2 core by electrochemical oxidation of the previously reported precursor [( Me2(OMe) TPA) 2 Fe III/IV (μ-O) 2 ](ClO 4 ) 3 (with Me2(OMe) TPA=tris(3,5-dimethyl-4-methoxypyridyl-2-methyl)amine) [72] . Combined Mössbauer and EXAFS data revealed that in [{( Me2(OMe) TPA)Fe IV } 2 (μ-O) 2 ] 4+ two low-spin ( S =1) Fe(IV)-centres are antiferromagnetically coupled and exhibit Fe–O and Fe–Fe distances of 1.78 and 2.73 Å, respectively. Cationic [{( Me2(OMe) TPA)Fe IV } 2 (μ-O) 2 ] 4+ could also be generated chemically, via the intermediate formation of an open-core [(O)Fe IV -O-Fe IV (OH)] 3+ complex cation, containing two S =1 Fe IV centres, by reacting the (μ-oxo)-diiron(III) precursor with H 2 O 2 in the presence of an acid [73] . Additionally, a new product with high-spin Fe IV S =2 and high-spin Fe III S =5/2 centres in a valence-localized [(O)Fe IV -O-Fe III (OH)] 2+ core was obtained by treating [( Me2(OMe) TPA) 2 Fe III Fe IV (μ-O) 2 ](ClO 4 ) 3 with hydroxide [74] . A comparative reactivity study of [{( Me2(OMe) TPA)Fe IV } 2 (μ-O) 2 ] 4+ , [(O)Fe IV -O-Fe IV (OH)] 3+ , [(O)Fe IV -O-Fe III (OH)] 2+ and the previously reported [72] S =1 [Fe IV =O] 2+ cations ( Fig. 5c ) showed that the terminal iron(IV) oxo units are at least three orders of magnitude more reactive than the ones with diamond cores [74] . The most potent C–H activator is the complex with an S =2 quintet ground state of the Fe=O moiety. Hence, for the first time, an experimental demonstration of increased reactivity of quintet oxoiron(IV) species over the corresponding triplet species was provided. Iron–nitrido intermediates in biology Iron-nitrido complexes, which are isoelectronic to iron–oxo complexes, are also considered as key intermediates in a number of important biological transformations. However, while a number of transient high-valent iron–oxo intermediates in the catalytic cycle of haem and non-haem enzymes have been identified and spectroscopically characterized [1] , [2] , [3] , [5] , [6] , [7] , [9] , [10] , [18] , direct evidence for the involvement of iron–nitrido intermediates in biology is lacking. Iron–nitride-mediated mechanistic postulates have nevertheless been motivated on the basis of indirect evidences that are obtained from various biochemical experiments [13] , [14] , [15] , [16] . For example, in the FeMo cofactor of the nitrogenase enzyme, the structure of which features seven iron centres and a single molybdenum centre held together by nine bridging sulphides and a carbide atom ( Fig. 7 ) [12] , [75] , dinitrogen reduction is proposed to occur at a single iron site [76] . Dinitrogen binds and is heterolytically cleaved at this iron site, which results in the release of ammonia and generation of Fe IV ≡N. However, alternative mechanisms involving molybdenum or polynuclear iron reactive sites have also been proposed in the literature [13] , [14] , [15] , [16] . Moreover, a related imidoiron(IV) porphyrin ( Fig. 7 ) species is postulated to be the reactive intermediate for cytochrome-P450-LM-3,4 catalysed N-atom transfer reactions [11] . 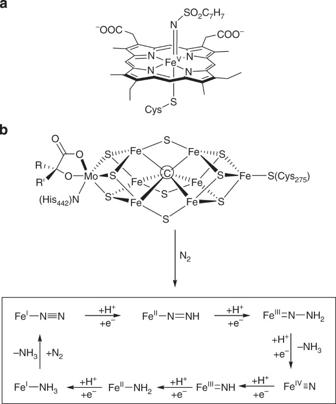Figure 7: Proposed structures of biological intermediates with iron–nitrogen multiple bonds. The proposed structures have inspired studies on model iron–nitrido and imido complexes. (a) Structure of the iron(IV) imido porphyrin intermediate that has been invoked for cytochrome-P450 catalysed nitrogen group transfer reactions11. (b) The iron molybdenum cofactor of the nitrogenase enzyme with a central carbide (C)12,75, and the proposed intermediates (scheme in the box) of the dinitrogen activation process occurring at a single iron site76. Figure 7: Proposed structures of biological intermediates with iron–nitrogen multiple bonds. The proposed structures have inspired studies on model iron–nitrido and imido complexes. ( a ) Structure of the iron(IV) imido porphyrin intermediate that has been invoked for cytochrome-P450 catalysed nitrogen group transfer reactions [11] . ( b ) The iron molybdenum cofactor of the nitrogenase enzyme with a central carbide (C) [12] , [75] , and the proposed intermediates (scheme in the box) of the dinitrogen activation process occurring at a single iron site [76] . Full size image Iron–nitrido model complexes To probe the possibility of the involvement of iron–nitrido intermediates in biological dinitrogen-reduction and atom-transfer reactions, bioinorganic chemists became interested in the synthesis and reactivity of model compounds involving high-valent nitridoiron moieties. Here we summarize the recent advances in this field with a focus on mono- and dinuclear complexes; thus, omitting the few rare examples of polynuclear iron–nitrido complexes [77] , [78] , [79] . The first high-valent nitridoiron complex was characterized in 1989, when Wagner and Nakamoto [80] photolysed a porphyrin-ligated Fe III azide complex [(TPP)Fe III (N 3 )] (TPP, tetraphenylporphinate anion) in a frozen matrix of dichloromethane at 30 K. The resulting matrix-stabilized nitrido complex [(TPP)Fe V (N)] exhibits a resonance Raman vibrational band centred at ν =876 cm −1 , which was assigned to the ν (Fe–N) stretching vibration ( Table 1 ). Labelling experiments with 57 Fe as well as 15 N allowed for the unambiguous assignment of this ν (Fe–N) band. Although no further spectroscopic characterization of the Fe V =N species was performed, the authors proposed—based on the relatively small force constant in comparison with the isoelectronic [(TPP)Mn(O)]—a d 3 high-spin ( S =3/2) rather than a low-spin S =1/2 electronic ground state for the nitridoiron(V) species [80] . The stabilization of the unusually high Fe V oxidation state in [(TPP)Fe V (N)] reflects the higher π-donating property of the nitrido ligand that stabilizes higher metal oxidation states; the isoelectronic [(TMP +• )Fe IV (O)] + complex [7] , [8] could only be stabilized as a d 4 oxoiron(IV) π-cation radical species. The higher π-donation from the nitrido ligand arises from the smaller effective nuclear charge (Z*) of nitrogen compared to oxygen [29] , which causes the N p orbitals to be better energetically matched with the valence d orbitals on Fe. Meyer et al . [81] reported the first high-yield synthesis of a nitridoiron(V) species by photolysis of trans -[(cy)Fe III (N 3 ) 2 ] + in frozen CH 3 CN; the reaction produced two species, which have been identified as the photo-reduced five-coordinate ferrous species, trans -[(cy)Fe II (N 3 )] + , formed via homolytic Fe–N 3 bond cleavage, and the photo-oxidized trans -[(N 3 )(cy)Fe V (N)] + , formed via homolytic N–N bond cleavage and N 2 evolution [81] . The high-valent Fe V species was identified unequivocally by its characteristic Mössbauer spectrum, with an isomer shift δ of −0.04 mms −1 and a quadrupole splitting Δ E Q of −1.90 mms −1 at 80 K ( Table 1 ) [81] . The Fe II complex was actually shown to be the major product of photolysis of the corresponding [(cy-ac)Fe III (N 3 )] + complex in solution (CH 3 CN at −35 °C) [40] , while the formation of the photo-oxidized Fe V complex [(cy-ac)Fe V (N)] + prevailed in a frozen matrix. Interestingly, the Mössbauer isomer shift δ of −0.04 mms −1 reported [40] , [81] for the pentavalent Fe ion in [(cy-ac)Fe V (N)] + and trans -[(N 3 )(cy)Fe V (N)] + is found to be similar to that of 0.01 mms −1 reported [40] for tetravalent Fe in [(cy-ac)Fe IV (O)] + and significantly more positive than the value reported for Collins' [(TAML)Fe V (O)] complex (−0.46 mms −1 ) [32] . This trend of higher isomer shifts in nitrido as compared with the corresponding oxo complexes has been explained [29] on the basis of higher covalency of the iron–nitrido bond (compared with the iron–oxo). The nitridoiron(V) species trans -[(N 3 )(cy)Fe V (N)] + and [(cy-ac)Fe V (N)] + have initially been reported to possess a high-spin d 3 , S =3/2, electronic ground state. However, in a subsequent in-depth spectroscopic and theoretical work, Aliaga-Alcalde et al . [82] concluded that [(cy-ac)Fe V (N)] + has an unusual orbitally degenerate S =1/2 ground state. Initially, the Fe–N stretch in [(cy-ac)Fe V (N)] + could not be identified in the infrared vibrational spectrum. However, by using synchrotron-based nuclear-resonant-vibrational-spectroscopy coupled to DFT, Petrenko et al . [83] identified the ν (Fe–N) band unambiguously at 864 cm −1 . Furthermore, the (photochemically inactive) ferric azide of the corresponding methylated cyclam ligand can be oxidized to yield [(Me 3 cy-ac)Fe IV (N 3 )] 2+ , which, in turn, is photochemically active. Accordingly, photolysis at 650 nm in frozen matrix yields another, yellow product, [(Me 3 cy-ac)Fe VI (N)] 2+ with one major component (73%) at δ =−0.29 mms −1 and Δ E Q =1.53 mms −1 in the Mössbauer spectrum [84] . This unusually low, negative isomer shift is consistent with a hexavalent Fe VI ≡N species. The assignment is further supported by a short Fe–N distance of 1.57 Å (determined by EXAFS), a complementary computational analysis, and a linear relationship between the isomer shifts and oxidation states in a series of complexes with similar iron complex core structures and varying formal oxidation states, ranging from +II to +VI (ref. 84 ). This is the first Fe VI coordination complex ever reported, with the ferrate anion FeO 4 2− being the only other known example of an Fe VI ion. However, just like all previous nitridoiron species, complex [(Me 3 cy-ac)Fe VI (N)] 2+ is only stable in cryogenic matrices and decomposes to a high-spin Fe III species on warming. In 2004, Betley and Peters [85] synthesized the first terminal Fe IV ≡N complex that is stable in solution at room temperature. By using a phenyl- tris -diisopropylphosphinoborate PhBP i Pr 3 − as the stabilizing tripodal chelate and lithium amide 2,3,5,6-dibenzo-7-azabicyclo[2.2.1]hepta-2,5-diene (dbabh) as the N-atom transfer reagent, the four-coordinate [( PhBP i Pr 3 )Fe IV (N)] could be obtained and thoroughly characterized by 1 H-, 31 P- and 15 N-NMR, Mössbauer and infrared spectroscopy in solution ( Table 1 ) [85] . An EXAFS analysis provided further insight into the molecular structure of [( PhBP i Pr 3 )Fe IV (N)] and revealed the unusually short Fe–N bond distance of 1.51–1.55 Å [86] . An X-ray diffraction analysis of the crystallized product remained elusive due to dimerization to a dinitrogen bridged Fe I /Fe I -dinuclear species on concentration change during solvent evaporation. This dimerization, a six-electron reaction mediated by two iron centres, is by itself a remarkable reaction. The observation of significant amounts of ammonia on treatment of [( PhBP i Pr 3 )Fe IV (N)] with protons and electrons is even more significant and lend credence to the involvement of similar intermediates during biological dinitrogen reduction. The structural characterization of Fe IV ≡N complexes by single-crystal X-ray diffraction was first accomplished in 2008. Photolysis of an N-anchored tris(carbene)-ligated azide complex [(TIMEN mes )Fe II (N 3 )] + (TIMEN mes =tris[2-(3-mesitylimidazol-2-ylidene)ethyl]amine) yielded the four-coordinate tetravalent [(TIMEN mes )Fe IV (N)] + as a purple crystalline material [87] . The spectroscopic fingerprint (infrared, 15 N NMR and Mössbauer spectroscopy) of [(TIMEN mes )Fe IV (N)] + is very similar to Peters' complex [( PhBP i Pr 3 )Fe IV (N)] ( Table 1 ). Even the crystallographically determined Fe–N distance of 1.526 Å in [(TIMEN mes )Fe IV (N)] + is (within the experimental error) identical to that of EXAFS-spectroscopically determined one in [( PhBP i Pr 3 )Fe IV (N)]. However, the geometries in these two nitrido complexes are markedly different. While the coordination polyhedron in the tris(phosphino)borate nitridoiron(IV) is best described as tetrahedral, the four-coordinate amine-anchored tris(carbene) nitride is trigonal pyramidal with the iron centre located approximately 0.4 Å above the plane of the carbene carbons. Also, while the axial nitride in [( PhBP i Pr 3 )Fe IV (N)] is relatively unprotected, the functionalization of the imidazole N3 nitrogens in the tris(carbene) of [(TIMEN mes )Fe IV (N)] + with sterically encumbering xylene and mesitylene groups places these substituents perpendicular to the tris(carbene)—iron plane; thus, creating a narrow cylindrical cavity, and effectively preventing bimolecular decomposition pathways. Moreover, the nitrido 15 N resonance in cationic [(TIMEN mes )Fe IV (N)] + ( δ =741 p.p.m. rel. to CH 3 NO 2 ) is considerably down-field shifted compared with the neutral [( PhBP i Pr 3 )Fe IV (N)] ( δ =572 p.p.m.) and, hence, is more similar to the nitrido ligand in trans -[(CF 3 COO)(cy)Mn V (N)] + (Mn V , d 2 , S =0) [88] . DFT calculations predict a diamagnetic {( x 2 − y 2 ) 2 ( xy ) 2 }{( z 2 ) 0 ( xz ) 0 ( yz ) 0 } electronic ground state, which is in agreement with the diamagnetic 1 H NMR spectra of these Fe IV ≡N complexes. The {( x 2 − y 2 ) 2 ( xy ) 2 }{( z 2 ) 0 ( xz ) 0 ( yz ) 0 } configuration also leads to an extreme asymmetric electron distribution around the Fe ion, which results in the largest quadrupole splitting parameters ever observed with Δ E Q values of more than 6 mms −1 ( Table 1 , Fig. 3 ). The S =0 ground state [85] , [87] of [(TIMEN mes )Fe IV (N)] + and [( PhBP i Pr 3 )Fe IV (N)] is, however, in stark contrast to the S =2 ground state of the [(TMG 3 tren)Fe IV (O)] 2+ complex [59] , [60] with an {( x 2 − y 2 ) 1 ( xy ) 1 ( xz ) 1 ( yz ) 1 ( z 2 ) 0 } electronic configuration ( Fig. 3 ). Although all three complexes possess a threefold symmetry, the strong antibonding character of the π*( xz , yz ) orbitals in [(TIMEN mes )Fe IV (N)] + and [( PhBP i Pr 3 )Fe IV (N)], which results in the inversion of the ( z 2 ) and ( xz ), ( yz ) levels, is likely due to differences in Z* between N and O that allow for better π-overlap to occur for Fe≡N multiple bond [29] . Scepaniak et al . [90] combined the ligand systems of Vogel et al . [87] and Betley and Peters [85] by using the phenyl- tris (1- tert -butylimidazol-2ylidene)borate (PhB( t BuIm) 3 − ), a boron-anchored tripodal tris(carbene) ligand system originally introduced by Fränkel et al . [89] Photolysis of [(PhB( t BuIm) 3 )Fe II (N 3 )] also yielded the corresponding diamagnetic Fe IV ≡N species, the complex [(PhB( t BuIm) 3 )Fe IV (N)], which was characterized by 1 H and 15 N NMR spectroscopy as well as electronic absorption spectroscopy, resonance Raman spectroscopy and single-crystal diffraction studies [90] . Similar to [(PhBP i Pr 3 )Fe IV (N)], this nitridoiron(IV) species possesses a pseudo-tetrahedral geometry with an S =0 electronic ground state. The reactivity of [(PhB( t BuIm) 3 )Fe IV (N)], however, is surprisingly different to that of [( PhBP i Pr 3 )Fe IV (N)]. While [(PhB( t BuIm) 3 )Fe IV (N)] reportedly does not react with protons and electrons, the carbene-based nitride engages in electrophilic reactions with phosphines, like Ph 3 P, yielding the phosphiniminato complex [PhB( t BuIm) 3 Fe II (NPPh 3 )], a rare example of a four-coordinate Fe II complex with a sharp S =2↔ S =0 spin-crossover transition at 78 K [91] . Most interestingly, the iron(IV) complex [(PhB( t BuIm) 3 )Fe IV (N)] could be oxidized with [Fe(Cp) 2 ]BAr F (with BAr F =tetrakis(3,5-bis(trifluoromethyl)phenyl)borate) to yield the corresponding pentavalent Fe V ≡N complex [(PhB( t BuIm) 3 )Fe V (N)] + , which is the first example of an Fe V ≡N that could be isolated and thoroughly characterized in solution and in solid state [92] . An X-ray diffraction study revealed overall similar bond metrics to its tetravalent precursor, with the most remarkable feature being the very short Fe–N bond distance of 1.502 Å in crystals of [(PhB( t BuIm) 3 )Fe V (N)]BAr F ( Table 1 ). The complex was further investigated by EPR and Mössbauer spectroscopy, supplemented by DFT calculations ( Table 1 ), thereby confirming the doublet ground state. Like Peters' Fe IV nitride [( PhBP i Pr 3 )Fe IV (N)], but not its Fe IV precursor, [(PhB( t BuIm) 3 )Fe IV (N)], the nitridoiron(V) complex reacts with protons (from water) under reductive conditions at −78 °C in tetrahydrofuran and evolves almost quantitative yields of NH 3 with concomitant formation of an Fe II species. Dinuclear model complexes As mentioned in the previous section, photolysis of Fe III azide complexes leads to the generation of a photo-oxidized Fe V terminal nitride species and a photo-reduced Fe II species. At ambient temperature, the Fe II and Fe V species react with each other to yield μ-nitrido-bridged Fe III /Fe IV complexes. Thus, via photolysis of [(Me 3 tacn)(Cl 4 cat)Fe III (N 3 )] (Me 3 tacn, 1,4,7-trimethyl-1,4,7-triazacyclononane; Cl 4 cat 2− , tetrachlorocatecholate) in solution at ambient temperature, Justel et al . [93] synthesized the nitrido-bridged dinuclear complex [(Me 3 tacn)(Cl 4 cat)Fe III (μ-N)Fe IV (Cl 4 cat)(Me 3 tacn)]. This mixed-valent diiron compound has two iron centres with distinct oxidation states of +III and +IV, which could be oxidized with bromine to yield the symmetrical Fe IV =N=Fe IV complex. Both species have been crystallographically characterized, but only the Fe IV /Fe IV species allowed for the unambiguous determination of the Fe IV –N bond distance of 1.703(1) Å within the Fe IV =N=Fe IV moiety. The total and residual electron densities of [(Me 3 tacn)(Cl 4 cat)Fe III (μ-N)Fe IV (Cl 4 cat)(Me 3 tacn)] were modelled with two disordered positions for the bridging nitrogen, implying that the core unit is not symmetrical and has two different Fe–N bond distances. In accordance with this model, the Mössbauer spectra of mixed-valent [(Me 3 tacn)(Cl 4 cat)Fe III (μ-N)Fe IV (Cl 4 cat)(Me 3 tacn)] showed two distinct Mössbauer doublets with isomer shifts at δ= 0.52 and 0.09 mms −1 , characteristic for octahedral high-spin Fe III and low-spin Fe IV ions, respectively ( Table 1 ). These results provide strong evidence for localized valencies at the iron centres of [(Me 3 tacn)(Cl 4 cat)Fe III (μ-N)Fe IV (Cl 4 cat)(Me 3 tacn)], in contrast to those of the nitrido-bridged diiron complex [(TPP)Fe 3.5 (μ-N)Fe 3.5 (TPP)], reported in 1976, where the excess electron is fully delocalized, resulting in formal oxidation states of 3.5 at both iron centres [94] . Remarkably, replacing one of the bidentate catecholate ligands in [(Me 3 tacn)(Cl 4 cat)Fe III (N 3 )] with the acetylacetonate derivative 1,3-diphenylpropane-1,3-dionate (Ph 2 acac − ), and photolysing a 1:1 mixture of [(Me 3 tacn)(Cl 4 cat)Fe III (N 3 )] and [(Me 3 tacn)(Ph 2 acac)Fe III (N 3 )], yields the asymmetric binuclear complex [(Me 3 tacn)(Ph 2 acac)Fe III (μ-N)Fe IV (Cl 4 cat)(Me 3 tacn)] without a crystallographically imposed inversion centre. Consequently, the mixed-valent complex [(Me 3 tacn)(Ph 2 acac)Fe III (μ-N)Fe IV (Cl 4 cat)(Me 3 tacn)] allows for the unambiguous determination of the Fe–N bond distances within the Fe III –N=Fe IV moiety at 1.785(7) Å and 1.695(7) Å, respectively. However, the difference in bond lengths is not as large as expected and is merely attributed to the varying radii of the iron ions in the different oxidation states. The Mössbauer spectrum of [(Me 3 tacn)(Ph 2 acac)Fe III (μ-N)Fe IV (Cl 4 cat)(Me 3 tacn)] is very similar to that of [(Me 3 tacn)(Cl 4 cat)Fe III (μ-N)Fe IV (Cl 4 cat)(Me 3 tacn)] ( δ= 0.60 and 0.04 mms −1 ; Table 1 ), showing localized valencies in the asymmetric mixed-valent complex [95] . In 1999, Meyer et al . [81] continued the investigation of high-valent nitrido species formation via photolysis of the corresponding azido complexes. Photolysis of trans -[(cy)Fe III (N 3 ) 2 ] + and cis -[(cy)Fe III (N 3 ) 2 ] + in solution at ambient temperatures resulted in the formation of binuclear μ-nitrido-bridged complexes [{ trans -(cy)Fe III (N 3 )}(μ-N){ trans -(cy)Fe IV (N 3 )}] 2+ and [{ cis -(cy)Fe III (N 3 )}(μ-N){ trans -(cy)Fe IV (N 3 )}] 2+ , respectively [81] . On the basis of EPR and applied-field Mössbauer spectroscopy ( Table 1 ), the total spin state ( S t ) in these mixed-valent complexes, S t =1/2 for trans/trans and S t =3/2 for trans/cis -isomer, was explained based on the assumption of strong antiferromagnetic coupling of an intermediate-spin Fe III ( S= 3/2 in trans/trans ), or a high-spin Fe III ( S =5/2 in trans/cis ) with a low-spin Fe IV ( S =1) metal centre and localized valencies in the [Fe IV =N–Fe III ] 4+ core [93] . Employing reactive complexes of abundant metals for synthesis, catalysis and energy supply is of great current interest. Selective functionalization of unactivated C–H bonds in organic compounds, for example, is a highly attractive strategy in organic synthesis, and the oxidation of methane and water are considered 'holy grails' in synthetic chemistry [96] . Similarly, energy-efficient production of ammonia is extremely important, as fertilizers generated from ammonia are responsible for sustaining one-third of Earth's population. A range of metalloenyzmes achieve these challenging tasks in biology by activating dioxygen and dinitrogen and using cheap and abundant first-row transition metals, like iron and manganese. Such reactions are carried out under ambient conditions with high efficiency and high stereospecificity. The recent results presented here from the bioinorganic chemistry community lend credence to the participation of high-valent oxo–ion and nitrido–iron complexes in the above-mentioned processes. Oxo and nitridoiron model complexes have now been synthesized using dioxygen or dinitrogen as the oxidant, via mechanisms reminiscent of the O 2 and N 2 activation process proposed in biology. Many of these complexes show intriguing reactivities, which in turn have provided vital insights into the modelled enzymatic reactions. Among the most significant conclusion of these studies is the observed activation of the model ferryl unit on axial ligand coordination trans to the oxo group. This has been attributed to strong electron donation from the axial thiolate ligand and explains the high reactivity of the natural thiolate-bound P450-I. Another important finding is the recently demonstrated [73] , [74] increased reactivity of the linear [(O)Fe IV -O-Fe III (OH 2 )] 2+ model complex, as compared with the ring-like [Fe IV 2 (μ-O) 2 ] 2+ core, that provides evidence for a comparable, more ring-opened form of Q with a terminal Fe IV =O unit as the active species in the reactivity of MMO. Additionally, although direct evidence for the involvement of oxoiron(V) intermediates in water oxidation is lacking in the literature, Kundu et al . [97] , has recently demonstrated a O–O bond formation reaction mediated by polynuclear oxoiron(IV) intermediates. Such a metal-mediated O–O bond formation step is considered to be the most critical part of dioxygen evolution in photosystem-II [98] . In N 2 activation and transformation chemistry, Lee et al . (ref. 99 ) have shown that many important intermediates in a variety of oxidation states of a hypothetical N 2 to NH 3 conversion cycle can be accommodated at a mononuclear iron site. More recently, Rodriguez et al . [100] have demonstrated the potassium-assisted cooperativity of three iron centres in the activation and cleavage of dinitrogen and subsequent generation of ammonia on reaction of the nitride species with dihydrogen. Unfortunately, the reactions exhibited by the model complexes are found to be non-catalytic, with activities falling far short of the activity of the biological catalysts. The low reactivity of the model complexes can be explained by the inability of synthetic chemists to exactly reproduce the biological ligand and protein environment. For example, even the ligand set of two histidines and one carboxylate, as observed in the first coordination sphere of non-haem oxygenases, is extremely difficult to synthesize and manipulate. Similarly, it has not yet been possible to generate an oxoiron(IV) porphyrin π-cation radical model complex with an axial thiolate ligand trans to the iron–oxo unit, as observed in Cpd-I of cytochrome-P450. Additionally, no iron-based model complexes mimicking the FeMo cofactor activity of the nitrogenase enzyme are known in the literature, and, as a result, the role of the postulated carbide ligand in dinitrogen activation is far from understood. Thus, new and innovative synthetic strategies are needed to generate superoxidized iron centres in ligand environments that better resemble the active site of the metalloenzymes. This goal may eventually lead to the development of iron-catalysed selective functionalization of organic compounds or ammonia synthesis by using cheap and accessible sources of dioxygen or dinitrogen under ambient conditions. How to cite this article: Hohenberger, J. et al . The biology and chemistry of high-valent iron–oxo and iron–nitrido complexes. Nat. Commun. 3:720 doi: 10.1038/ncomms1718 (2012).